Viruses as new agents of organomineralization in the geological record Viruses are the most abundant biological entities throughout marine and terrestrial ecosystems, but little is known about virus–mineral interactions or the potential for virus preservation in the geological record. Here we use contextual metagenomic data and microscopic analyses to show that viruses occur in high diversity within a modern lacustrine microbial mat, and vastly outnumber prokaryotes and other components of the microbial mat. Experimental data reveal that mineral precipitation takes place directly on free viruses and, as a result of viral infections, on cell debris resulting from cell lysis. Viruses are initially permineralized by amorphous magnesium silicates, which then alter to magnesium carbonate nanospheres of ~80–200 nm in diameter during diagenesis. Our findings open up the possibility to investigate the evolution and geological history of viruses and their role in organomineralization, as well as providing an alternative explanation for enigmatic carbonate nanospheres previously observed in the geological record. Microbial mats represent one of Earth’s earliest ecosystems [1] , [2] . However, due to diagenetic effects during rock lithification and the possible abiotic pathways for carbonate formation, the biogenic origin of ancient putative microbial mats is often controversial [3] . The study of modern microbial mats provides new insights into the microbial contribution to mineralization processes, and act as analogues to help understand mineralization processes that occurred in the past [4] , [5] . In these mats, microbes mediate the formation of mineral layers, typically carbonates, and in doing so they enhance their own preservation potential in the geological record; this process has been called organomineralisation [5] , [6] , a term that includes both microbially-induced and microbially-influenced mineralization. Cell walls, sheaths and extracellular polymeric substances (EPSs) are thought to be the main templates for mineral precipitation [6] , [7] , yet the role of viruses in organomineralization has largely been ignored despite the fact that viruses have been shown to be widespread in marine and terrestrial ecosystems [8] and more specifically in modern microbial mats [9] . Here we show how viruses influence organomineralization in a living microbial mat from the hypersaline lake Lagoa Vermelha, Brazil, where sulfate-reducing bacteria are already known to mediate dolomite formation [10] , and high-Mg calcite is known to precipitate on prokaryotic cell walls [11] . The data presented here are obtained from living mats collected from the natural lake setting (NLS) and from simulated diagenetic experiments (SDEs), in which mats were stored in dark, anoxic conditions for 6 months to 3 years, mimicking diagenetic conditions at the water–sediment interface. These experiments allowed us to trace the changes in abundance and morphology of viruses and their hosts both in their living state and after their mineralization, which is essential if such biosignatures are to be recognized in the geological record. Metagenomics Metagenomic analyses conducted on viral nucleic acids extracted from a living microbial mat from the hypersaline lake Lagoa Vermelha, Brazil ( Supplementary Fig. 1 ) revealed that a minor fraction of all high-quality reads are annotated ( Supplementary Fig. 2a ). These sequences are related to a total of 585 viral strains, the majority of which (~90%) are based on dsDNA, whereas only a small fraction belongs to ssDNA ( Fig. 1 ). We also found some RNA viral groups; however, the method used is specific for DNA amplification, so we cannot exclude the possibility of annotation artifacts here. The main hosts of the viruses are prokaryotes (that is, bacteria and archaea; Supplementary Fig. 2 ). Most viral strains belonged to bacteriophage families Siphoviridae and Myoviridae , which are non-enveloped, tailed viruses, ranging in size from 50–100 nm, but we also identified the presence of a relevant number of archaeoviral strains (viruses infecting archaea) belonging to families Fuselloviridae , Lipothrixviridae and Bicaudaviridae , plus nucleocytoplasmic large DNA viruses, such as Mimiviridae , displaying large capsids (>400 nm) and infecting eukaryotes. Virophages, that influence the infection success of other large viruses, such as Mimiviridae , were also present. 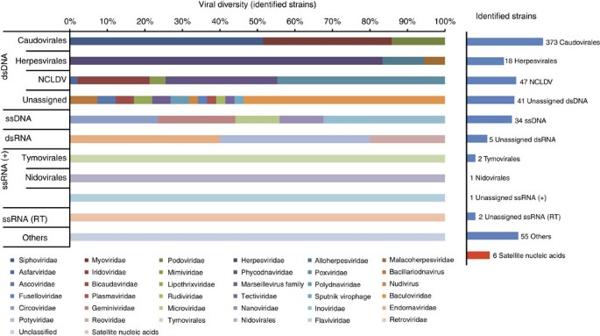Figure 1: Metagenomic analysis revealing the composition of the viral assemblages in the microbial mat. The total number of viral strains belonging to a specific order is shown on the right; when no specific order was identified, viral strains were grouped as ‘unassigned.’ Identified viral families are shown on the left, with the number of strains in each family as a percentage of the total number of strains per each order. Figure 1: Metagenomic analysis revealing the composition of the viral assemblages in the microbial mat. The total number of viral strains belonging to a specific order is shown on the right; when no specific order was identified, viral strains were grouped as ‘unassigned.’ Identified viral families are shown on the left, with the number of strains in each family as a percentage of the total number of strains per each order. Full size image Microscopy High-resolution imaging of the NLS microbial mat reveals abundant non-mineralized ~60–150-nm-sized particles that exhibit capsid-like structures that are often icosahedral ( Figs 2a,b and 3d ), consistent with Siphoviridae and Myoviridae morphology. Some of these virus-like particles are clearly associated with prokaryotic cell walls ( Supplementary Fig. 3 ), whereas other nano-sized particles (nanospheres) possess spheroidal outer envelopes ( Fig. 2b ). The large envelopes of some entities could be artifacts generated from sample preparation. However, although we cannot rule out the possibility of nano-sized organic debris, in depth image analyses indicate that most of these particles are different from those previously reported as artifacts [12] . 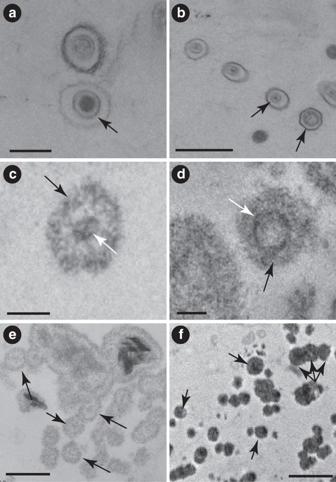Figure 2: Bright-field TEM images showing the morphology and distribution of virus-like particles in the living microbial mat under natural lake conditions (a–d) and after simulated diagenesis (e–f) from Lagoa Vermelha. (a) Virus-like particle characterized by an icosahedral capsid-like structure (black arrow). Scale bar, 200 nm. (b) Virus-like particles. Black arrows point to the capsid-like structure in each case. Scale bar, 500 nm. (c) First stage of theamMg-Si mineralization process of the icosahedral capsid-like structure (black arrow); white arrow points to the viral DNA inside. Scale bar, 100 nm. (d) Second stage of theamMg-Si mineralization process of a virus-like particle (black arrow) showing its icosahedral capsid-like structure (white arrow). Scale bar, 100 nm. (e) Early mineralization of virus-like particles showingamMg-Si permineralized capsid-like structures (arrows). Scale bar, 200 nm. (f)amMg-Si permineralized virus-like particles occurring as single entities and chains (examples arrowed). Scale bar, 500 nm. Figure 2: Bright-field TEM images showing the morphology and distribution of virus-like particles in the living microbial mat under natural lake conditions ( a – d ) and after simulated diagenesis ( e – f ) from Lagoa Vermelha. ( a ) Virus-like particle characterized by an icosahedral capsid-like structure (black arrow). Scale bar, 200 nm. ( b ) Virus-like particles. Black arrows point to the capsid-like structure in each case. Scale bar, 500 nm. ( c ) First stage of the am Mg-Si mineralization process of the icosahedral capsid-like structure (black arrow); white arrow points to the viral DNA inside. Scale bar, 100 nm. ( d ) Second stage of the am Mg-Si mineralization process of a virus-like particle (black arrow) showing its icosahedral capsid-like structure (white arrow). Scale bar, 100 nm. ( e ) Early mineralization of virus-like particles showing am Mg-Si permineralized capsid-like structures (arrows). Scale bar, 200 nm. ( f ) am Mg-Si permineralized virus-like particles occurring as single entities and chains (examples arrowed). Scale bar, 500 nm. 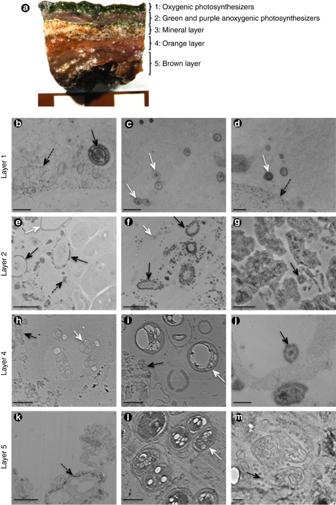Figure 3: Vertical transect of the microbial mat from Lagoa Vermelha under natural lake conditions showing the different microbial and mineral components. (a) Cross-section of a microbial mat showing stratified layers of carbonate precipitation alternating with microbial community layers. Numbers on the right side correspond to the sampled organic layers. (b–m) Bright-field TEM images showing the different mineralization stages occurring in the successive layers in the living microbial mat: (b–d) layer 1, which is mainly constituted by oxygenic photosynthetic organisms38, did not show any evidence of (per)mineralization, but cyanobacteria (see the intact thylakoid membranes inside the cell (b, black arrow)), fibrillar EPS (dashed arrows) and virus-like particles (white arrows) were all common. Layer 2 is dominated by phototrophic sulphide oxidizers38and displayed the early (amorphous Mg-Si) permineralization stages (e–g) occurring within EPS (black dashed arrow) and around some prokaryotic cells (black arrows), whereas algal cell walls and other prokaryotes remained non-mineralized (white arrow). Virus-like particles were still recognizable (g). Note that early permineralization corresponds to the oxic–anoxic transition in the mat. (h–j) Layer 4 showed an increase inamMg-Si precipitates (black arrows), while prokaryotes containing intracellular inclusions remained non-mineralized (white arrows). Early mineralization of virus-like particles also occurred in this layer (j). (k–m) Layer 5 showed abundant prokaryotic cells containing inclusions (white arrow), likely SRB as they dominated the deepest part of the microbial mat38. Empty cells were mineralized and displayed more crystalline parts (dashed arrow). Some virus-like particles remained non-mineralized (black arrow). Scale bar, 2 μm (e–f,h–i,k), 1 μm (l), 500 nm (b–c,g), 200 nm (d,j,m). Full size image Figure 3: Vertical transect of the microbial mat from Lagoa Vermelha under natural lake conditions showing the different microbial and mineral components. ( a ) Cross-section of a microbial mat showing stratified layers of carbonate precipitation alternating with microbial community layers. Numbers on the right side correspond to the sampled organic layers. ( b – m ) Bright-field TEM images showing the different mineralization stages occurring in the successive layers in the living microbial mat: ( b – d ) layer 1, which is mainly constituted by oxygenic photosynthetic organisms [38] , did not show any evidence of (per)mineralization, but cyanobacteria (see the intact thylakoid membranes inside the cell ( b , black arrow)), fibrillar EPS (dashed arrows) and virus-like particles (white arrows) were all common. Layer 2 is dominated by phototrophic sulphide oxidizers [38] and displayed the early (amorphous Mg-Si) permineralization stages ( e – g ) occurring within EPS (black dashed arrow) and around some prokaryotic cells (black arrows), whereas algal cell walls and other prokaryotes remained non-mineralized (white arrow). Virus-like particles were still recognizable ( g ). Note that early permineralization corresponds to the oxic–anoxic transition in the mat. ( h – j ) Layer 4 showed an increase in am Mg-Si precipitates (black arrows), while prokaryotes containing intracellular inclusions remained non-mineralized (white arrows). Early mineralization of virus-like particles also occurred in this layer ( j ). ( k – m ) Layer 5 showed abundant prokaryotic cells containing inclusions (white arrow), likely SRB as they dominated the deepest part of the microbial mat [38] . Empty cells were mineralized and displayed more crystalline parts (dashed arrow). Some virus-like particles remained non-mineralized (black arrow). Scale bar, 2 μm ( e – f , h – i , k ), 1 μm ( l ), 500 nm ( b – c , g ), 200 nm ( d , j , m ). Full size image In both the SDE mat and the mineral layers of the NLS mat, mineralized nano-particles (~80–200 nm in diameter) are common ( Figs 2c–f and 4 ). Epifluorescence microscopy analyses (using either a single DNA stain or the CARD-FISH methodology, specific to bind RNA) confirmed the presence of nucleic acids within the early stage mineralized nano-particles ( Supplementary Fig. 4 ), ruling out the possibility that these virus-like particles are merely nano-sized minerals or minerals precipitated on proteins. These data also reveal the large numerical dominance of such particles over prokaryotes in the mat ( Supplementary Fig. 5 ). The early stages of mineralization are observed from the dysoxic part of the NLS mat, where capsid-like structures are still recognizable ( Figs 2c–e and 3 ). 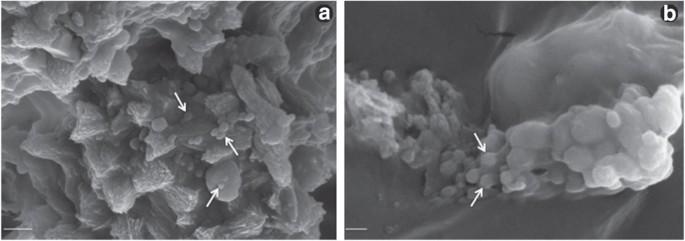Figure 4: SEM photomicrographs showing the presence of nanospheres in mineral layers within the Lagoa Vermelha microbial mat under natural conditions. (a) Carbonate-mineralized nanospheres (for example, white arrows) located in the mineral layers before HF–HCl acid digestion. Scale bar, 1 μm. (b) Some nanospheres display a hexagonal shape (arrows). Scale bar, 300 nm. Figure 4: SEM photomicrographs showing the presence of nanospheres in mineral layers within the Lagoa Vermelha microbial mat under natural conditions. ( a ) Carbonate-mineralized nanospheres (for example, white arrows) located in the mineral layers before HF–HCl acid digestion. Scale bar, 1 μm. ( b ) Some nanospheres display a hexagonal shape (arrows). Scale bar, 300 nm. Full size image Long-term exposure to anoxic conditions in the SDE mats resulted in a greater abundance of both mineralized and non-mineralized virus-like particles outside prokaryote cells, and a clear increase in the number of permineralised particles—occurring either as single entities or aggregates ( Figs 2e–f and 5 ). Fully mineralized Mg-carbonate nanospheres in the mineral layers of the NLS mat also retain virus-like morphology ( Fig. 2d ). Elemental analysis of the virus-like particles indicates that initial permineralisation occurs as amorphous Mg-Si ( am Mg-Si) phases ( Supplementary Fig. 6 ), whereas NanoSIMS analysis of the same area shows a direct correlation between organic material and silicate mineralogy ( Fig. 6 ). This suggests that the virus-like particles are primary nucleation sites for mineral precipitation. Anoxic conditions appear to enhance the mineralization potential of both the prokaryotic cells and of the virus-like particles themselves. Un-mineralized organic particles with similar size and morphology to directly adjacent mineralized prokaryotes ( Fig. 5 ) indicate that mineralization is not indiscriminate, suggesting that only infected cells become mineralized. 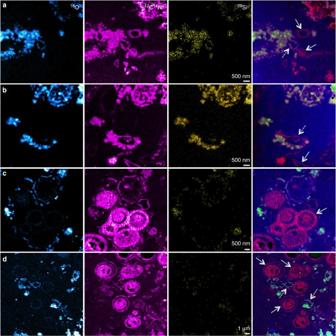Figure 5: NanoSIMS secondary ion images showing16O−,12C14N−,28Si−and RGB composites of the same region. The CN signal indicates organic material, whereas O and Si indicate mineralized material. The RGB composites (composed of12C14N−,16O−and12C2−in the RGB channels, respectively) help to show where elements are colocated. (a) This region (the same region inFig. 6) features un-mineralized organic material (arrows) directly adjacent to the mineralized material with similar morphology (dashed arrow). Field of view=6 μm. (b) This region shows a partially mineralized cell-like feature (dashed arrow) and un-mineralized organic material (arrow). The image was acquired with slightly lower resolution to capture more signal, hence the stronger contrast in the Si image. Field of view=6 μm. (c) Some prokaryote cells remain largely un-mineralized (arrow). Field of view=8 μm. (d) Large un-mineralized prokaryote cells (arrows) adjacent to smaller mineralized prokaryote cells (dashed arrows). Field of view=15 μm. Figure 5: NanoSIMS secondary ion images showing 16 O − , 12 C 14 N − , 28 Si − and RGB composites of the same region. The CN signal indicates organic material, whereas O and Si indicate mineralized material. The RGB composites (composed of 12 C 14 N − , 16 O − and 12 C 2 − in the RGB channels, respectively) help to show where elements are colocated. ( a ) This region (the same region in Fig. 6 ) features un-mineralized organic material (arrows) directly adjacent to the mineralized material with similar morphology (dashed arrow). Field of view=6 μm. ( b ) This region shows a partially mineralized cell-like feature (dashed arrow) and un-mineralized organic material (arrow). The image was acquired with slightly lower resolution to capture more signal, hence the stronger contrast in the Si image. Field of view=6 μm. ( c ) Some prokaryote cells remain largely un-mineralized (arrow). Field of view=8 μm. ( d ) Large un-mineralized prokaryote cells (arrows) adjacent to smaller mineralized prokaryote cells (dashed arrows). Field of view=15 μm. 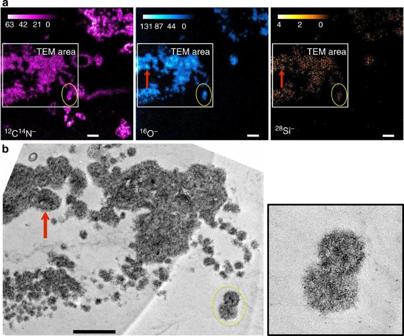Figure 6: Correlative NanoSIMS and TEM images of virus mineralization within EPS in the microbial mat after 3 years of simulated diagenesis. (a) NanoSIMS ion maps of identical analysis areas show one-to-one correlation between organic material (12C14N−) and silicate mineral phases (16O−and28Si−). (b) TEM image shows virus morphology and exact correlation to the boxed portion of the NanoSIMS chemical maps. Circled viruses are the same in all images (and enlarged in the boxed TEM image). A second possible rounded virus (arrow) likely corresponds to a more advanced stage in the mineralization process because of its larger size. Scale bar, 500 nm. Full size image Figure 6: Correlative NanoSIMS and TEM images of virus mineralization within EPS in the microbial mat after 3 years of simulated diagenesis. ( a ) NanoSIMS ion maps of identical analysis areas show one-to-one correlation between organic material ( 12 C 14 N − ) and silicate mineral phases ( 16 O − and 28 Si − ). ( b ) TEM image shows virus morphology and exact correlation to the boxed portion of the NanoSIMS chemical maps. Circled viruses are the same in all images (and enlarged in the boxed TEM image). A second possible rounded virus (arrow) likely corresponds to a more advanced stage in the mineralization process because of its larger size. Scale bar, 500 nm. Full size image Amorphous Mg-Si precipitates have previously been reported in carbonate environments, and are always associated with microbial activity [13] , [14] , [15] . It has also been demonstrated that am Mg-Si enhances fossilization, and is commonly found in the rock record [13] . The authigenesis of am Mg-Si phases is, however, poorly understood, with previous work suggesting that am Mg-Si layers in microbialites are a replacement of a primary mineral phase [14] . In contrast, our data indicate a primary origin for these am Mg-Si phases. Previous studies have established the role of cell walls and EPS as nucleation sites for am Mg-Si precipitates, leading to prokaryote fossilization [13] , [15] . Like EPS, the viral capsid is composed of proteins containing reactive carboxyl and amine groups [16] , [17] that are known to have a key role in cation binding [6] and thus, can act as a template for mineralization [18] . Indeed, the material properties of viral capsids are utilized in biomimetics where viruses are used as scaffolds for mineralization [19] . Thus, we here propose to add viruses to the list of templates for am Mg-Si mineralization within microbial mats. With continued diagenesis in calcium carbonate-rich environments, progressive Ca incorporation and subsequent replacement of much of the am Mg-Si material by carbonate likely leads to the common geological occurrence of calcified bacterial cells, carbonate nanospheres and am Mg-Si phases [13] , [14] , [15] . This is indeed observed in both our diagenetic experiments and within the lithified layers in Lagoa Vermehla itself ( Fig. 4 ). Furthermore, as evident from the epifluorescence data, viruses are by far the most abundant biological component, outnumbering prokaryotes by two orders of magnitude ( Supplementary Fig. 5 ), and therefore might logically be expected to be the main drivers of organomineralisation in this environment. Here we propose a new model in which viruses have a key role in organomineralization processes ( Fig. 7 ). Viruses infect their hosts by attaching themselves to specific receptors on prokaryotic cell walls, then injecting their genetic material inside the cell. Metagenomic analyses conducted in the microbial mat revealed a great diversity of viruses ( Fig. 1 ). In addition, most of the sequences we found belong to unknown strains and did not match with currently available databases. Our findings confirmed the presence of viral genes potentially incorporated by prokaryotes (CRISPRs) inhabiting the Lagoa Vermelha mat (see Supplementary Fig. 7 ), providing supporting evidence that viral infections occur in both bacteria and archaea. In infections characterized by lytic cycles, viral replication results in the host cell bursting, with the consequent release of the newly formed viruses along with cellular debris. A minority of these viruses (1–5%) infect other prokaryote cells [20] , but a large majority remain free in the mat, and represent the largest fraction of nano-sized particles that can undergo degradation or, under specific conditions, mineralization processes. In the investigated system, these viruses along with the cellular debris undergo am Mg-Si permineralization. The am Mg-Si phase may be progressively replaced by Mg-carbonates, concomitant with the formation of successive mineral layers within the microbialite. 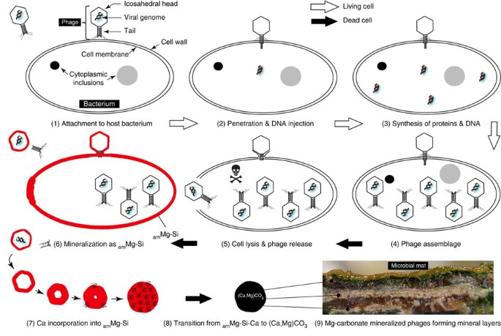Figure 7: Model showing the evolution from virus attachment to a prokaryotic cell through to virus mineralization. (1) Virus attachment to specific receptors on prokaryotic cell walls; (2) injection of genetic material inside the cell by tail contraction; (3) disruption of the host’s normal metabolism leading to manufacture of viral products; (4) virus assemblage within the infected cell; (5) viruses released outside the prokaryotic cell after cell lysis; (6) Mg-Si permineralization of viruses concomitant with prokaryotic cells in dysoxic conditions; (7) incorporation of calcium into Mg-Si polygons and spheres; (8) replacement ofamMg-Si-Ca phases by Mg-carbonate; (9) mineralized viruses in microbial mat carbonate layers occurring as distinct nanometer-scale spheroids. Figure 7: Model showing the evolution from virus attachment to a prokaryotic cell through to virus mineralization. (1) Virus attachment to specific receptors on prokaryotic cell walls; (2) injection of genetic material inside the cell by tail contraction; (3) disruption of the host’s normal metabolism leading to manufacture of viral products; (4) virus assemblage within the infected cell; (5) viruses released outside the prokaryotic cell after cell lysis; (6) Mg-Si permineralization of viruses concomitant with prokaryotic cells in dysoxic conditions; (7) incorporation of calcium into Mg-Si polygons and spheres; (8) replacement of am Mg-Si-Ca phases by Mg-carbonate; (9) mineralized viruses in microbial mat carbonate layers occurring as distinct nanometer-scale spheroids. Full size image Our data also suggest an alternative origin for carbonate nano-sized spheres found throughout the geological record [21] . Such nanospheres were initially attributed to ‘nannobacteria’ or dormant bacteria [22] , but these interpretations are controversial because nanospheres are thought to be too small to house all of the necessary DNA, RNA and plasmids contained within prokaryotes [23] . More recently, nanospheres have been interpreted as either bacterial fragments, EPS [23] or membrane vesicles [24] and it has been suggested that these components are significant contributors to the biomineralization process [25] . In contrast, our correlative high-resolution imaging and metagenomic analyses provide new and mutually supporting evidence that mineralized nm-sized spheres in a microbial mat have a biological signature and are derived from viruses and the results of their infections. Our results indicate that viruses, numbering in the order of 10 11 g −1 ( Supplementary Fig. 5 ), are crucially important in nucleation processes that control the mineralization of microbial mats. The ability to identify viruses in the geological record has wide ranging implications because viruses are important agents of genetic exchange and mortality for all life forms, and have fundamental roles in global biogeochemical cycles [20] , [26] . Although viruses are known for their pathogenic effect, viral infections can also stimulate the metabolism, the immunity and promote the evolution of their hosts [27] . They have important roles in oceans, infecting photosynthetic organisms and controlling primary production [28] , and act as primary agents of mortality of prokaryotes in deep-sea sediments [29] . Moreover, viruses serve as gene reservoirs that allow their hosts to adapt to changing ecological niches [28] . Viruses may have been instrumental in promoting the evolution of early microbial ecosystems on Earth. This is particularly pertinent here given that viruses are so abundant within a microbial mat, one of Earth’s most primitive and enduring ecosystems. Here we propose the criteria for correctly identifying fossilized viruses in the rock record that include: (1) a size of ~20–200 nm (>99% of all known viruses); (2) the association of nano-sized spheres with larger fossil cells or cell-like pseudomorphs; (3) the association of these nanospheres with critically tested microbially induced sedimentary structures [30] or other microbial fabrics; (4) the presence of organic nanospheres after acid dissolution of the mineral fraction. As the morphologies of viral capsids are quite variable, the identification of a specific virus-like morphology (for example, polygonal outlines) can support the criteria above, but it is not a pre-requisite. Additional criteria can be far more problematic, such as the presence of a tail in viral-like particles (VLPs), which is unlikely to be preserved in ancient examples, and could be easily mimicked by abiotic mineral growths. As with any ancient putative biological structure, multiple lines of mutually supporting evidence would be required for a confident interpretation of nanospheres as fossil viruses, but data similar to those reported here would allow the rejection of the hypothesis of an inorganic and abiotic origin for these spherical mineral growths [31] . This will be no easy task, but the new findings reported in this study opens up the potential to identify viruses in the geological record and understand more about their geological and evolutionary history. Simulated diagenesis experiments The microbial mat was placed in a small dark anoxic chamber where oxygen was replaced by nitrogen for a duration of 6 months to 3 years. The comparison between the natural sample and the one that had undergone the simulated diagenesis experiment was carried out using electron microscopy (scanning electron microscopy (SEM) and transmission electron microscopy (TEM), see below) and a microelectrode. The latter was used for real-time measurement of pH in the upper 30 mm of the mat, following the methodology of Visscher et al . [32] Under natural conditions, pH values in similar microbial mats fluctuate between <6.5 and >9 in a day – night cycle, with the lowest pH values observed during nighttime [33] . After experimental diagenesis in our study, the pH values were constant throughout the mat with an average value of 8.6. Electron microscopy showed an increase in Mg-carbonate crystals as well as an increase in am Mg-Si nanospheres. The latter were observed in the area containing no visible Mg-carbonate crystals for TEM preparations. Close to Mg-carbonate crystals, prokaryotes embedded in EPS contained Ca in addition to Mg and Si ( Supplementary Fig. 2 ), thereby suggesting a progressive Ca incorporation into metastable am Mg-Si phases before conversion to stable Mg-carbonates. Sample preparation for TEM and NanoSIMS Before staining, samples were fixed in 2% glutaraldehyde in 0.1 M cacodylate buffer (CB) at pH 7.4 and at room temperature for 1 hour, washed three times in CB, and postfixed in 1% osmium tetroxide in CB for one hour at room temperature. After three washes in CB, the material was embedded in 2.5% agarose and dehydrated before inclusion in Epon resin. Sections (70 nm for electron microscopy) were cut on a Leica ultramicrotome using a diamond knife (Diatome). Sections for electron microscopy were transferred onto carbon-coated films on copper grids or onto single slot grids coated with Formvar films. Ultrathin sections were stained for 10 min in 1% uranyl acetate in water. Transmission electron microscopy TEM observations were performed with a Phillips CM100 transmission electron microscope (Paris-Sud University and Zurich University) and Phillips CM120 (Claude Bernard Lyon 1 University), and digital image processing was applied. Elemental analyses were performed using EDAX genesis 4000 on a CM120 STEM (University of Zurich). Scanning electron microscopy Microbial mat samples were fixed in 2% glutaraldehyde, then platinum coated before imaging with a Jeol JSM 6400 SEM. (University of Zurich, Switzerland). CARD-FISH and epifluorescence counting of VLPs and cells Microbial mat samples were analysed under epifluorescence microscopy using SYBR Gold as a stain [34] for epifluorescence counting of VLPs and cells. Briefly, VLPs and cells were detached from the extracellular matrix by physical and chemical treatments and then mounted on 0.02 μm aluminium oxide membrane filters (Whatman Anodisc) before staining with SYBR Gold. For CARD-FISH analyses, samples were fixed with 2% buffered formalin and hybridized with labelled probes for differential counts of bacteria and archaea [35] . NanoSIMS High-resolution elemental mapping was performed on the same thin sections used for TEM. Secondary ion images were acquired using the CAMECA NanoSIMS 50 ion microprobe at The University of Western Australia. Following TEM analysis, the sample was coated with 10 nm of gold to ensure conductivity at high voltage. A Cs + primary beam was used to sputter the negative ion species 16 O − , 12 C 2 − , 12 C 14 N − , 28 Si − secondary electrons. The primary beam was focused to a beam diameter of ~50 nm in high-resolution mode, with a beam current of ~0.1 pA. As there were no significant isobaric interferences, it was not necessary to tune the mass spectrometer to high mass resolution. Before imaging, a thin layer of Cs was deposited on the regions of interest using a low-energy primary beam. This novel approach allows the sample to achieve a steady-state of secondary ion yield without high-energy presputtering, which would otherwise destroy the fragile ultrathin section [36] . Images were acquired at a resolution of 256 × 256 pixels by rastering the beam over an area of 6 × 6 μm, 8 × 8 μm or 15 × 15 μm, with a dwell time of 20 ms per pixel. The relatively short dwell time ensured that the delicate ultrathin sections were not destroyed by the ion beam. The sections would typically ‘burn through’ after two or three images were acquired. Hence, it was not possible to collect data using both the Cs + and O − ion sources on the same sections, meaning that the distribution of cations such as Ca and Mg could not be mapped from the same sections as 16 O − , 12 C, 14 N − , 28 Si − . The data were corrected for a detector dead-time of 44 ns on the individual pixels. Metagenomics Viral particles were recovered from microbial mat samples including the different layers by means of physical and chemical treatments. Briefly, 50 g of microbial mat were diluted 10-fold and distributed in 15 ml tubes, then treated with tetrasodium pyrophosphate, followed by sonication and centrifugation [34] . Pellets were washed three times following the same procedure and supernatants were collected before filtering onto 0.2 μm membrane filters to remove cell debris. The eluate was treated with DNase I for 4 h to remove contaminating nucleic acids, then mounted on 0.02 μm aluminium oxide membrane filters (Whatman Anodisc). Viral nucleic acids were extracted following the manual protocol described by Sambrook et al . [37] with some modifications. Briefly, each filter was added with 20 mM EDTA, 10% SDS and proteinase K before incubation at 56 °C for one hour. Viral DNA was purified through two subsequent phenol–chloroform treatment steps followed by isopropanol precipitation. After fluorimetric quantification, replicate samples of viral DNA ( n =3) were amplified by GenomiPhi V2 kit (GE Healthcare) and pooled together. Pooled replicates were purified using Wizard PCR and Gel Clean-up kit (Promega). Before pyrosequencing, potential contamination due to prokaryotic and eukaryotic DNA was checked in the viral DNA sample by PCR targeting 16S and 18S rRNA genes and gel electrophoresis analysis. After having ruled out the presence of contaminating prokaryotic or eukaryotic DNA, the sample was sequenced using a 454 FLX Titanium platform (Macrogen Inc., Korea). Sample processing for metagenomic analyses of viral DNA was performed by the Microbial and Molecular Ecology laboratory of the Polytechnic University of Marche. To remove sequencing artifacts and low-quality sequences, reads were analysed by using the UCLUST service provided by the MG-RAST v3 server [39] . The same pipeline was used to analyse functional assignments, for example, presence of CRISPR sequences. Afterwards, cleaned sequences were submitted to MetaVir [40] . Viral metagenomes were annotated using the tool GAAS [41] , comparing reads against the RefSeq database with an E-value threshold of 10 −5 and normalizing the results for the genome length of each taxon. Taxonomic affiliations and average viral genome size were computed and, to investigate viral diversity, automated phylogenies for specific marker genes and viral families were constructed. To bypass biases related to preferential amplification of specific DNA structures by the phi29 polymerase included in the MDA kit used [42] , we counted the number of identified viral strains instead of the sequences affiliated to them. Richness of viral strains, affiliation of viruses to families and nucleic acid structure were determined in this way. When such affiliations were not possible to ascertain, strains were collected into the respective ‘unassigned’ groups. How to cite this article: Pacton, M. et al . Viruses as new agents of organomineralization in the geological record. Nat. Commun. 5:4298 doi: 10.1038/ncomms5298 (2014). Accession codes: Metagenomic data have been deposited in the Metavir database ( http://metavir-meb.univ-bpclermont.fr/ ) under Project name ‘Lagoa Vermelha’.